Ultrafast spin exchange-coupling torque via photo-excited charge-transfer processes Optical control of spin is of central importance in the research of ultrafast spintronic devices utilizing spin dynamics at short time scales. Recently developed optical approaches such as ultrafast demagnetization, spin-transfer and spin-orbit torques open new pathways to manipulate spin through its interaction with photon, orbit, charge or phonon. However, these processes are limited by either the long thermal recovery time or the low-temperature requirement. Here we experimentally demonstrate ultrafast coherent spin precession via optical charge-transfer processes in the exchange-coupled Fe/CoO system at room temperature. The efficiency of spin precession excitation is significantly higher and the recovery time of the exchange-coupling torque is much shorter than for the demagnetization procedure, which is desirable for fast switching. The exchange coupling is a key issue in spin valves and tunnelling junctions, and hence our findings will help promote the development of exchange-coupled device concepts for ultrafast coherent spin manipulation. Control of coherent spin precession in ferromagnets is currently a popular topic due to its importance in magnetic recording and spintronic devices [1] , [2] , [3] , [4] , [5] , [6] . The search for non-thermal excitation mechanisms motivates extensive research to overcome the disadvantages of thermal ones. The main idea is to utilize the interaction between magnetization and photo-excited carriers that are selectively optical pumped, where the recombination time of photocarriers is much shorter than the heat diffusion process. A promising approach is through ferromagnetic–antiferromagnetic (FM–AFM) exchange coupling, as small modulation of the exchange-coupling strength might lead to notable changes in magnetic properties [7] , [8] . Recent studies demonstrated that short laser pulses can introduce non-thermal spin reorientation and dynamics in AFM materials much faster than in FM materials [9] , [10] . But the question is still open whether it is possible to drive FM magnetization at the speed of AFM materials through FM–AFM exchange across heterostructure interface. In this article, optical excitation of spin precession is investigated in Fe/CoO exchange-coupled heterostructure with time-resolved magneto-optic Kerr effect (TRMOKE). Photo-excited charge-transfer processes in AFM CoO layer create a strong transient exchange-coupling torque on FM Fe layer through FM–AFM exchange coupling. The efficiency of spin precession excitation is significantly higher and the recovery is notably faster than the demagnetization procedure. The precession amplitude peaks around room temperature and with external magnetic field competitive to the magnetic anisotropy field, indicating that this efficient excitation mechanism originates from the modulation of the uniaxial magnetic anisotropy K u induced by the FM/AFM exchange coupling. Our results will help promote the development of low-energy consumption magnetic device concepts for fast spin manipulation at room temperature. Description of ultrafast spin exchange-coupling torque The observed ultrafast spin precession excitation is described by a modified Landau–Lifshitz–Gilbert (LLG) equation with an additional torque term: where γ is gyromagnetic ratio, M is the magnetization, H eff is the effective magnetic field, α is the Gilbert damping constant, denotes the instant spin exchange-coupling torque, and Δ H ex ( t ) is the change of FM–AFM exchange field H ex by modulation of uniaxial exchange anisotropy K u , as discussed further below. The geometry of instant spin exchange-coupling torque is illustrated in Fig. 1 . 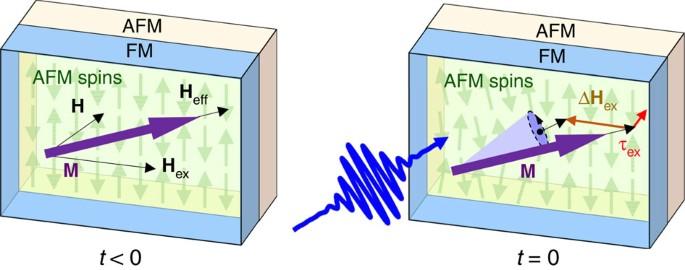Figure 1: Illustration of photo-excited spin exchange-coupling torque. Att<0, the magnetizationM(purple arrow) in the Fe layer aligns along the effective field directionHeff(black arrow).Hdenotes the external magnetic field, andHexis the field established by FM–AFM exchange coupling. Att=0, the 400-nm pump pulse (blue arrow) generates photo-excited carriers in the CoO layer, which leads to the reorientation of AFM spins (green arrows). This modifies the exchange coupling, ΔHex(brown arrow), causing a change of the effective field direction. Then the exchange-coupling torque(red arrow) forms, which triggers the precession ofM. Figure 1: Illustration of photo-excited spin exchange-coupling torque. At t <0, the magnetization M (purple arrow) in the Fe layer aligns along the effective field direction H eff (black arrow). H denotes the external magnetic field, and H ex is the field established by FM–AFM exchange coupling. At t =0, the 400-nm pump pulse (blue arrow) generates photo-excited carriers in the CoO layer, which leads to the reorientation of AFM spins (green arrows). This modifies the exchange coupling, Δ H ex (brown arrow), causing a change of the effective field direction. Then the exchange-coupling torque (red arrow) forms, which triggers the precession of M . Full size image Structure and static magnetic properties The Fe/CoO and Fe thin films are deposited on MgO(001) substrates by molecular beam epitaxy (MBE) at room temperature (see Methods) [7] . The thickness of CoO and Fe layers are 3 nm and 4 nm, respectively. All of the samples are covered with a 3-nm-thick MgO protection layer, and the epitaxial relation is CoO[110]//Fe[100]. Reflection high-energy electron diffraction patterns reveal the high-quality, epitaxial growth of the CoO and Fe films (see Supplementary Fig. 1 ). Longitudinal MOKE measurements are carried out with external magnetic field applied along the Fe [100] and [010] directions ( Fig. 2a , right). The easy-axis hysteresis loops show perfect squareness, indicating the single domain of the Fe film (see Supplementary Fig. 2 and Supplementary Note 1 ). 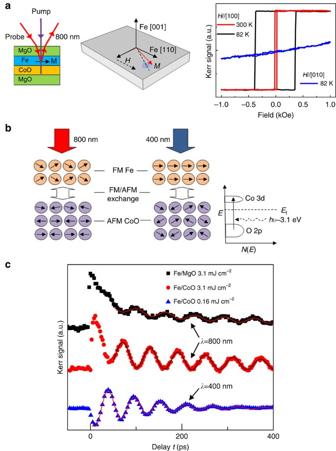Figure 2: Experimental design and observation of ultrafast exchange-coupling torque. Schematic of TRMOKE measurement geometry, depiction of magnetization precession and longitudinal hysteresis loops (a). Two pump strategies to optically excite the spin precession (b), where the black arrows represent the magnetic moments. Optical charge-transfer transition in CoO is depicted. TRMOKE results from Fe/MgO (black squares) and Fe/CoO (red circles) with pump-pulse intensity 3.1 mJ cm−2, and Fe/CoO (blue triangles) with pump intensity 0.16 mJ cm−2(c). The solid lines represent fits of equation (2). Figure 2: Experimental design and observation of ultrafast exchange-coupling torque. Schematic of TRMOKE measurement geometry, depiction of magnetization precession and longitudinal hysteresis loops ( a ). Two pump strategies to optically excite the spin precession ( b ), where the black arrows represent the magnetic moments. Optical charge-transfer transition in CoO is depicted. TRMOKE results from Fe/MgO (black squares) and Fe/CoO (red circles) with pump-pulse intensity 3.1 mJ cm −2 , and Fe/CoO (blue triangles) with pump intensity 0.16 mJ cm −2 ( c ). The solid lines represent fits of equation (2). Full size image Observation of ultrafast spin exchange-coupling torque Coherent spin precessions in the Fe layers are investigated by pump-probe TRMOKE (see Methods) in a canted magnetization configuration where the magnetic field ( H ) is applied along Fe [110] direction, as depicted in Fig. 2a . In equilibrium, the magnetization is along an effective field H eff , which is the sum of H , the demagnetizing field H d and the anisotropy field H a . The incident pump pulses induce a transient field H tr , and the magnetization M starts to precess around H tr . When H tr has vanished, the vector M is away from its original equilibrium orientation along H eff . Therefore, it starts to precess around H eff as depicted in Fig. 2a . In general, the amplitude will show a resonance-type dependence on an external field, and the position and frequency of the resonance are determined by the external field and the magnetic parameters such as the values of the various anisotropy constants. Two strategies of pump are employed in the measurements to investigate the optical excitation mechanisms: First, the more intense pump pulses ( λ =800 nm, 3.1 mJ cm −2 ) are used to modulate the FM order of Fe layer as shown in Fig. 2b (left) since the CoO layer is almost transparent to 800-nm light [11] ; Second, the weaker pump pulses ( λ =400 nm, 0.16 mJ cm −2 ) are utilized to mainly affect the AFM order of CoO as depicted in Fig. 2b (right). All TRMOKE measurements are performed after field cooling the sample. The TRMOKE result from Fe/MgO heterostructure is displayed in Fig. 2c (black squares) with pump-pulse fluence 3.1 mJ cm −2 and magnetic field H =2 kOe at room temperature. The sudden rise and decay of Kerr signal indicates the demagnetization process. Meanwhile, the magnetization starts to precess around the equilibrium direction in a damped circling way described by LLG equation [12] , [13] . The measured Kerr signal can be well-fitted by the following equation where parameters A , τ , f and ϕ are the amplitude, magnetic relaxation time, frequency and initial phase of the magnetization precession mainly along the polar direction, respectively. Here, a and t 0 are related to the background signal owing to the slow recovery of magnetization after fast demagnetization by the pump pulses, which happens mainly along the longitudinal direction. Figure 2c (red circles) shows TRMOKE result from Fe/CoO(3 nm)/MgO structure with the same excitation condition as the measurement on Fe/MgO (black squares). We note that the background amplitude a remains unchanged, while the amplitude of coherent spin precession A is enhanced. This shows that the AFM CoO layer improves the efficiency of optically excited coherent spin precession. The key finding here is that pronounced spin precession is still observed with much lower pump-pulse energy 0.16 mJ cm −2 at 400-nm wavelength, as shown in Fig. 2c (blue triangles). Moreover, the TRMOKE data reveal the absence of obvious demagnetization and slow recovery of M . The instant pronounced spin precession points towards an ultrafast non-thermal excitation process in the AFM CoO layer as depicted in Fig. 2b (right) and discussed further below. Furthermore, the magnetic relaxation time τ decreases from 330 ps (red circles) to 100 ps (blue triangles) in Fe/CoO with 400-nm pump pulses, which is desirable for fast switching. To determine the origin of the optical excitation mechanism, temperature and field-dependent TRMOKE measurements are carried out ( Fig. 3 ). 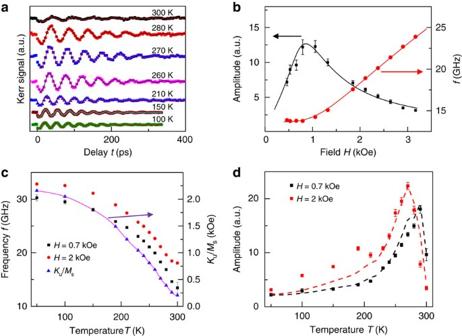Figure 3: Temperature and field-dependent TRMOKE studies. TRMOKE results from Fe/CoO at different temperaturesT(a), where the solid lines are fits of equation (2). Spin precession amplitudeA(black squares) and frequencyf(red circles) as a function ofH(b). The solid lines are simulations. The arrows indicate the proper y-axis for the different plots (b,c). Temperature dependence offfor two different fields (c). The derivedKu/MSis also plotted (blue triangles) and linked with spline cubic analysis fitting. Temperature dependence ofAfor two different fields (d), where solid lines represent simulated results. Error bar ofAis estimated by the deviation of fitting with equation (2). Figure 3: Temperature and field-dependent TRMOKE studies. TRMOKE results from Fe/CoO at different temperatures T ( a ), where the solid lines are fits of equation (2). Spin precession amplitude A (black squares) and frequency f (red circles) as a function of H ( b ). The solid lines are simulations. The arrows indicate the proper y-axis for the different plots ( b , c ). Temperature dependence of f for two different fields ( c ). The derived K u / M S is also plotted (blue triangles) and linked with spline cubic analysis fitting. Temperature dependence of A for two different fields ( d ), where solid lines represent simulated results. Error bar of A is estimated by the deviation of fitting with equation (2). Full size image Temperature- and field-dependent studies Figure 3a presents TRMOKE results ( λ =400 nm, H =2 kOe) with pump-pulse intensity 0.16 mJ cm −2 at different temperatures T , where the absence of demagnetization peak is observed. Figure 3b displays the precession frequency f (red circles) and amplitude A (black squares) as a function of H at room temperature. The frequency f is well-fitted with LLG equation (red curve) to derive the magnetic anisotropies (see Supplementary Note 2 and Supplementary Table 1 ) [8] . The simulation of A versus H (black curve), where A is assumed to be proportional to the equilibrium direction change by modulation of K u (Δ K u =165 Oe × M S ) (refs 14 , 15 , 16 ) (see Supplementary Note 3 ), agrees quite well with the experimental data. M S is the saturation magnetization. Furthermore, K u increases significantly with decreasing T , while M S remains unchanged (see Supplementary Figure 3 and Supplementary Note 1 ), as shown by the blue triangles in Fig. 3c . The derived K u / M S behaves similarly like f (red circles and black squares) as a function of T . The FM–AFM exchange coupling establishes an extra preference of magnetization alignment in Fe, where the FM spins favour perpendicular alignment with the frozen AFM spins due to the spin flop coupling between them. As the number of frozen AFM spins in CoO grows with lower T , the FM/AFM exchange coupling builds up, which leads to an increase of K u and hence f rises with lower T as shown in Fig. 3c . Figure 3d displays the precession amplitude A as a function of T for different H . The amplitude A peaks around 270 K ( H =2 kOe) and 290 K ( H =0.7 kOe), when H is approximately equal to the anisotropy field H a . At higher temperatures, A drops sharply similar to K u / M S , because the AFM order in CoO is greatly diminished above 270 K, since the temperature is close to its Neel temperature ( ∼ 290 K) and the FM/AFM exchange coupling becomes weaker. Therefore the uniaxial anisotropy K u is small compared with H when approaching room temperature. This behaviour is similar to the peak shown in Fig. 3b . As T decreases, K u enhances H a , which requires a stronger H to compete with H a , hence the generated transient torque and amplitude A decrease. As a result, the peak in A shifts to lower T and becomes broader at higher fields, which agrees well with the simulation based on the modulation of K u (dashed curves). Therefore, the origin of this efficient excitation mechanism with 400-nm pump pulses has to be the modulation of magnetic anisotropy constant K u . The modulation of K u also sheds light on the difference between the two optical excitation strategies, 800-nm versus 400-nm wavelength pump pulses. On one hand, the CoO layer is almost transparent to light with λ =800 nm, as its bandgap is ∼ 2.5 eV (ref. 11 ). Therefore, the 800-nm pump pulses mainly excite hot electrons in the FM Fe layer as depicted in Fig. 2b (left) which also modulate the FM–AFM exchange coupling and hence K u . This leads to improvement of spin precession excitation efficiency as compared with Fe/MgO thin film ( Fig. 2c ). Ju. et al . [17] reported that in the exchange-coupled NiFe/NiO bilayer the photo-excited hot electrons in the FM layer partially diffuse to the interface and slightly modulate the interface AFM order. The authors called this process an ‘ultrafast unpinning of the exchange bias’ [17] . The authors also note that the bulk magnetic structure of NiO is frozen [17] . This is markedly different from the phenomenon observed here, which we assume here to modulate the AFM order in the CoO layer. Photon-induced interband transitions occur in bulk CoO at λ =455 nm (2.73 eV) (see Supplementary Note 4 ). Hence the near-gap, 400-nm pump photons excite charge-transfer transitions from O 2p-band to Co 3d-band that is partially occupied with minority spins, as depicted in Fig. 2b (ref. 18 ). This promotes the nearest-neighbour FM exchange interaction [19] , which modulates the AFM order in the CoO layer. Similarly, Duong et al . [20] reported ultrafast manipulation of AFM order in NiO. Photoexcitation of NiO leads to ultrafast reorientation of Ni 2+ spins due to change of the magnetic anisotropy [20] . The variance of AFM order in CoO layer notably modulates the FM/AFM exchange coupling and K u , since the coupling between Fe and CoO is a long-range interaction [21] . This leads to a change of the effective field direction, as depicted in Fig. 1 , causing a transient torque on the ferromagnetic magnetization and thus leads to significant enhancement of the excited FM spin precession. We call this process an ‘ultrafast spin exchange-coupling torque’, which is markedly different from the ultrafast unpinning process due to hot electrons in the FM layer. For the ultrafast spin exchange-coupling torque, the carrier excitation is instant on photoexcitation, thus the AFM modulation is fast. In addition, the exchange interaction between Fe FM spins and CoO AFM spins are very strong and the modulation of this exchange interaction is fast. Among the magnetic interactions, the spin exchange-coupling interaction has the largest energy and thus the shortest time scale. This process is also repeatable many times without any thermally induced degradation. Larger magnetization precession may be obtained with shorter wavelengths, thereby enhancing (reducing) the absorption in the CoO (Fe) layer, which will also lower the thermal load (larger heat capacity of CoO) allowing the application of higher pump-pulse power. To investigate the duration of this fast FM–AFM exchange torque, simulations of real-time magnetization precession are carried out from LLG equation. The observed pronounced coherent spin precession starts right at t =0, indicating a sudden change of equilibrium direction caused by Δ K u . We assume that the reduction of K u (165 Oe × M S ) happens instantly at t =0, followed by an exponential recovery process with time constant τ r , as shown by the blue curve in Fig. 4 . With τ r =40 ps, the simulated time evolution of magnetization (red curve) agrees quite well with the probed Kerr signal (black dots), since the TRMOKE signal is proportional to the polar component of magnetization precession. Shorter or longer τ r leads to mismatch in the oscillation phase (See Supplementary Fig. 4 ). The fast recovery from photo-excited transitions might be due to the strong carrier-phonon interaction, which results in non-radiative and phonon-assisted carrier recombination [22] . Moreover, the recovery time of the instant photo-induced exchange-coupling torque is much faster than the cooling time from demagnetization, which can promote novel device concepts for fast spin manipulation. 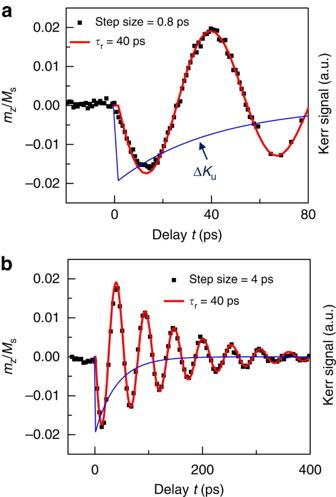Figure 4: Simulation of real-time magnetization precession. Measured Kerr signal change (black squares), simulated polar magnetization component (red curve) and assumed modulation ofKu(blue curves) as a function of time delayton short (a) and long (b) time scales. Figure 4: Simulation of real-time magnetization precession. Measured Kerr signal change (black squares), simulated polar magnetization component (red curve) and assumed modulation of K u (blue curves) as a function of time delay t on short ( a ) and long ( b ) time scales. Full size image In summary, the efficiency of spin precession excitation by laser pulses is significantly improved by inserting an AFM CoO layer in Fe/MgO heterostructure, which establishes the uniaxial magnetic anisotropy K u along Fe [100] direction. The modulation of K u by laser pump pulses generates a fast exchange-coupling torque to the FM Fe magnetization. The transient torque is enhanced at temperatures where K u varies significantly and with external magnetic fields comparable to the magnetic anisotropy fields. The excitation is much more efficient with 400-nm pump pulses via photo-excited charge-transfer processes in AFM CoO layer than modulating the FM order of Fe via generation of hot electrons with 800-nm-wavelength pulses. The recovery time of the exchange-coupling torque is ∼ 40 ps, much faster than the cooling time from demagnetization. Our results will help promote the development of low-energy consumption magnetic device concepts for fast spin manipulation at room temperature. Sample fabrication The Fe/CoO thin films are grown on the MgO(001) substrate in an ultrahigh vacuum chamber with MBE. The MgO(001) substrate with a miscut angle <0.5° is prepared by annealing at 600 °C for 30 min. The AFM CoO thin films are grown by a reactive deposition of Co under an oxygen pressure of 2 × 10 −6 torr. A 4-nm-thick Fe film is then grown epitaxially on top of the CoO film at room temperature. All samples are covered with a 3-nm-thick MgO protection layer. As a control group, Fe thin films are grown directly on the MgO substrate with MBE at room temperature. MOKE measurements In the longitudinal MOKE studies, we measured the FM magnetization of Fe layer by irradiating the sample with p-polarized light and detecting the s-component of the reflected light with a photodiode. The external magnetic field is applied in-plane along the Fe [100] or [010] directions from 80 K to above room temperature. Time-resolved MOKE measurements We performed TRMOKE measurements in a pump-probe set-up, where the intensity ratio of the pump to probe pulses is set to be about 6:1. The probe ( λ =800 nm) utilizes the MOKE technique with crossed polarizers and incident angle ∼ 40° to investigate the transient magnetic state change along longitudinal and polar directions. The intense pump pulses (3.1 mJ cm −2 ) are generated by a Ti/sapphire amplifier laser system delivering 150-fs pulses at 800-nm wavelength with a repetition rate of 1 kHz. The 400-nm pump pulses (0.16 mJ cm −2 ) are generated by frequency-doubling the 800-nm pulses (200 fs) from a 250-kHz Ti/sapphire laser system in a beta barium borate (BBO) crystal. Data analysis and simulations The TRMOKE raw data is fitted using the built-in non-linear-fit function of Origin 8.5 software with expression programmed as equation (2). The uncertainties of A and f are provided by the software from least squares fitting. Least square methods are also programmed with Matlab 2014 and used to fit the change of f and A as functions of H with Supplementary Equations 1 and 3 (see Supplementary Note 3 ), where the uncertainties of anisotropy fields are estimated through error propagation method. To simulate the real-time magnetization precession in Fig. 4 , LLG equation is written numerically in Supplementary Equations 4 and 5 , with very small time interval Δ t =0.2 ps (see Supplementary Note 5 ). The evolution of y and z magnetization components with time is derived through iteration, which is programmed with Matlab 2014. How to cite this article: Ma, X. et al . Ultrafast spin exchange-coupling torque via photo-excited charge-transfer processes. Nat. Commun. 6:8800 doi: 10.1038/ncomms9800 (2015).